Highly active deficient ternary sulfide photoanode for photoelectrochemical water splitting The exploration of photoanode materials with high efficiency and stability is the eternal pursuit for the realization of practically solar-driven photoelectrochemical (PEC) water splitting. Here we develop a deficient ternary metal sulfide (CdIn 2 S 4 ) photoanode, and its PEC performance is significantly enhanced by introducing surface sulfur vacancies, achieving a photocurrent density of 5.73 mA cm −2 at 1.23 V vs. RHE and 1 Sun with an applied bias photon-to-current efficiency of 2.49% at 0.477 V vs. RHE. The experimental characterizations and theoretical calculations highlight the enhanced effect of surface sulfur vacancies on the interfacial charge separation and transfer kinetics, which also demonstrate the restrained surface states distribution and the transformation of active sites after introducing surface sulfur vacancies. This work may inspire more excellent work on developing sulfide-based photoanodes. The efficient utilization of solar energy may afford a renewable route to alleviate the energy and environmental issues caused by the increasing consumption of fossil fuels [1] . Apart from photovoltaics (PV), which convert solar energy into electricity, photoelectrochemical (PEC) water splitting is recognized as another promising strategy and attracts particular interest for storing solar energy into the chemical bonds of hydrogen fuel, which can be further released and utilized in fuel cells or internal combustion engines [2] , [3] . To achieve high solar to hydrogen (STH) conversion efficiencies in practical PEC cells, the choice of electrode materials, especially the photoanodes, is of great importance in the consideration of the sluggish, multistep, proton-coupled electron transfer kinetics of water oxidation on photoanodes surfaces [4] . Up to now, some of the most promising semiconductors employed as photoanodes include α-Fe 2 O 3 [5] , BiVO 4 [6] , Ta 3 N 5 (TaON) [7] , [8] , and TiO 2 [9] . However, no semiconductor so far fully satisfies all the stringent requirements for practical application, including the high STH efficiency, robust stability in aqueous electrolytes, and low cost for scalable module manufacturing, which renders the design of satisfactory photoanode materials still challenge. Other than making efforts on the current photoanodes materials, exploring novel semiconductors and employed as photoanodes maybe supply a new route. The optimal tandem PEC cell ideally is consisted of a photoanode with a bandgap of ~2.0 eV and a photocathode with a bandgap of ~1.2 eV to achieve the highest STH efficiency and unassisted water splitting [10] . Therefore, the semiconductors that possess proper bandgaps and band-edge potentials theoretically have the potential to be employed as photoanodes. Among others, metal sulfides have long been the topic of research, especially photocatalytic applications due to their suitable electronic bandgaps, exposed active sites, diverse and adjustable chemical structures [11] . However, apart from the factor of photochemical photocorrosion, which can be dramatically suppressed by the usage of sacrificial agents or surface decoration of passive layers [12] , [13] , [14] , the metal sulfides directly employed as photoanodes usually exhibit low photoinduced electron–hole separation efficiencies and sluggish surface water oxidation kinetics [15] , [16] , [17] , [18] , which limits the application of metal sulfides-based photoanodes. The defects in metal sulfide, especially for introducing sulfur vacancies, are evidenced as an effective strategy to enhance the photocatalytic and PEC properties [19] , [20] , [21] , [22] . The trap states introduced by sulfur vacancies can act as capture centers to enable charge carrier separation. Besides, the charge density of metal sulfide can also be significantly increased after introducing sulfur vacancies, which results in the shortening of depletion width and enhancement for the band bending for hole collection [23] . Moreover, recent research reveals that the adjacent atoms after introducing sulfur vacancies turn into the active sites for oxygen evolution reaction (OER), which can facilitate the surface water oxidation kinetics [24] . Benefit from all these reasons, we consider that introducing sulfur vacancies into metal sulfides-based photoanodes may also be an efficient strategy to improve their PEC performance. Herein, we develop a deficient ternary metal sulfide (CdIn 2 S 4 ) and employ it as a photoanode. We introduce sulfur vacancies to the CdIn 2 S 4 photoanode through mild annealing treatment, and the PEC performance of the CdIn 2 S 4 photoanode is significantly enhanced, revealing superior photocurrent density and applied bias photon-to-current efficiency (ABPE) compared to other up-to-date promising single photon absorbers. In addition, the effects of sulfur vacancies on the PEC performance and charge transfer kinetics are systematically elucidated by experimental characterizations and theoretical calculations. Specifically, the surface sulfur vacancies can restrain the surface states (SS) distribution on the CdIn 2 S 4 photoanode, which supplies an approach to adjusting the potentials at the semiconductor/electrolyte interface. Synthesis and physicochemical characterizations The synthetic protocol of the CdIn 2 S 4 photoanode with sulfur defects is illustrated in Fig. 1a , which involves two steps, i.e., hydrothermal treatment and subsequent annealing with an Ar/H 2 flow. Introducing heteroatoms or vacancies is usually more easily achieved under higher temperatures [25] . Therefore, the phase stability of the CdIn 2 S 4 under different annealing temperatures is first investigated. The powder X-ray diffraction (PXRD) patterns of the final products are shown in Fig. 1b and all the diffractions are well indexed to cubic CdIn 2 S 4 and FTO except for the product annealed at 550 °C, where the impurity phase of CdS appears as labeled by the asterisks. The evolution of the atomic coordination environment involved in as-prepared products at different temperatures is monitored using electron spin resonance (ESR) spectra (Fig. 1c ), which yields a g value of 2.004 that is assigned to the sulfur vacancy [26] . The upshift of S 2 p X-ray photoelectron spectra (XPS) of V s -CIS-500 further confirms the appearance of sulfur vacancy (Fig. 1d ) [24] , which is also validated by the Cd 3 d and In 3 d peaks shifting to lower binding energy to compensate the charge nonequilibrium (Supplementary Fig. 1 ). The peak position of O 1 s in V s -CIS-500 is nearly identical to that in pristine CdIn 2 S 4 , which illustrates the existence form of O should be surface hydroxyls (Supplementary Fig. 2 ). Besides, apart from the intensities of the ESR signals, the photocurrent of the products also reveals a positive correlation with the temperature but V s -CIS-550 (Supplementary Fig. 3 ). Thus, we consider that the V s -CIS-500 maybe possess the optimal PEC performance. The microstructure of V s -CIS-500 is investigated by scanning electron microscopy (SEM, Fig. 1e ), which exhibits plate-shaped geometry and reveals nearly no changes compared with that of the pristine CdIn 2 S 4 nanocrystals (Supplementary Fig. 4 ), indicating that the introduction of sulfur vacancies does not affect its morphology. The energy-disperse X-ray spectroscopy (EDS, Supplementary Fig. 5 ) confirms that the Cd, In, and S atoms distribute uniformly across the V s -CIS-500 nanoplate, also indicative of its structural stability during annealing treatment. Besides, the morphology of V s -CIS-500 is reconstructed according to the Bravais–Friedel–Donnay–Harker (BFDH) theory (inset of Fig. 1e ) [27] , and further surface energy calculations reveal that the ( \(0\overline 1 1\) ) crystal plane truncated with In and S atoms is the dominant exposed plane (see details in Supplementary Note 1 ). The formation energies of sulfur vacancies in all possible chemical potentials are calculated as well, which illustrate that the formation of sulfur vacancies is a thermodynamically endothermic process and ( \(0\overline 1 1\) ) is energetically the most feasible crystal plane to generate surface sulfur vacancies under all possible chemical potentials (see details in Supplementary Note 2 ). Thus, we consider that surface sulfur vacancies in the ( \(0\overline 1 1\) ) crystal plane is mainly responsible for the PEC performance changes of the CdIn 2 S 4 photoanode. The selected area electron diffraction (SAED, Supplementary Fig. 6 ) illustrates the single-crystal characteristic of V s -CIS-500, and the high-angle annular dark-field (HAADF) image (Fig. 1f ) further confirms the dominant ( \(0\overline 1 1\) ) crystal plane, as well as shows the existence of surface sulfur vacancies as marked by the circle. Moreover, the theoretical atomic structure of ( \(0\overline 1 1\) ) truncated with In and S atoms matches well with the HAADF-STEM image (inset of Fig. 1f ), which also corresponds to above surface energy calculation results. To further elucidate the effect of surface sulfur vacancies on the electronic structures of CdIn 2 S 4 nanocrystals, we performed Coulomb interaction corrected density functional theory (DFT + U ) calculations. As depicted in Fig. 1g , shallow trap states mainly consisted of S 3 p orbitals generate, which maybe contributes to enhanced photoabsorption or improve interfacial electron transfer processes. More importantly, the generation of surface sulfur vacancies results in the charge accumulation on the adjacent Cd and In atoms (Fig. 1h ), which may act as highly active sites for chemisorption of the intermediates during the OER, and facilitates the surface water oxidation kinetics. Fig. 1: Synthesis and characterizations of S deficient CdIn 2 S 4 nanocrystals. a The schematic diagram for the synthetic procedure of the CdIn 2 S 4 nanocrystals with sulfur vacancies. b PXRD patterns. c ESR spectra. d Core-level XPS spectra of S 2 p for CdIn 2 S 4 and V s -CIS-500. e The SEM image of V s -CIS-500. Inset is the reconstructed shape based on the BFDH theory. f The HADDF-STEM image of V s -CIS-500. Inset is the atomic structure of CdIn 2 S 4 ( \(0\overline 1 1\) ) with In and S as truncated atoms. g The density of states for CdIn 2 S 4 bulk and CdIn 2 S 4 ( \(0\overline 1 1\) ) with surface sulfur vacancies. h Different charge density image for the CdIn 2 S 4 ( \(0\overline 1 1\) ) with surface sulfur vacancies (isosurface set at 0.04e Bohr −3 ); yellow and cyan regions represent electron accumulation and depletion, respectively. Full size image PEC performance of CdIn 2 S 4 and V s -CIS-500 photoanodes The PEC performance of CdIn 2 S 4 and V s -CIS-500 photoanodes was investigated with a conventional three-electrode cell. The J–V plots obtained using AM 1.5 G illumination reveal that the photocurrent density of the V s -CIS-500 photoanode is greatly enhanced, achieving a value of 5.73 mA cm −2 at 1.23 V vs. RHE, and corresponds to a ~6 times increase compared with that of the pristine CdIn 2 S 4 photoanode (Fig. 2a ). 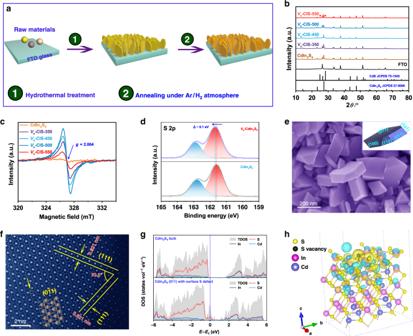Fig. 1: Synthesis and characterizations of S deficient CdIn2S4nanocrystals. aThe schematic diagram for the synthetic procedure of the CdIn2S4nanocrystals with sulfur vacancies.bPXRD patterns.cESR spectra.dCore-level XPS spectra of S 2pfor CdIn2S4andVs-CIS-500.eThe SEM image ofVs-CIS-500. Inset is the reconstructed shape based on the BFDH theory.fThe HADDF-STEM image ofVs-CIS-500. Inset is the atomic structure of CdIn2S4(\(0\overline 1 1\)) with In and S as truncated atoms.gThe density of states for CdIn2S4bulk and CdIn2S4(\(0\overline 1 1\)) with surface sulfur vacancies.hDifferent charge density image for the CdIn2S4(\(0\overline 1 1\)) with surface sulfur vacancies (isosurface set at 0.04e Bohr−3); yellow and cyan regions represent electron accumulation and depletion, respectively. 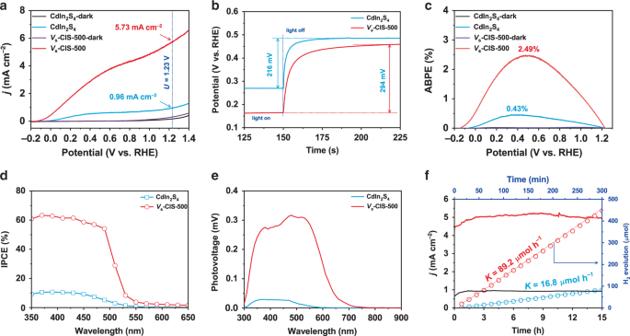Fig. 2: Photoelectrochemical performance. aCurrent–voltage (J–V) plots measured in 0.35 M Na2SO3and 0.25 M Na2S mixed solution (pH = 12.5) under dark and AM 1.5 G, 100 mW cm−2illumination with a scan rate of 10 mV s−1.bOpen-circuit voltages of CdIn2S4andVs-CIS-500 photoanodes were recorded in 0.5 M Na2SO4solution (pH = 7) in the dark and under illumination.cABPE measured with a two-electrode cell for water splitting in 0.35 M Na2SO3and 0.25 M Na2S mixed solution (pH = 12.5) under dark and AM 1.5 G, 100 mW cm−2illumination.dIPCE measured at 0.6 V vs. RHE under monochromatic light irradiation.eSPV spectra of CdIn2S4andVs-CIS-500 nanoparticles.fLong-term stability test, as well as experimental and theoretical H2evolution, were measured in 0.35 M Na2SO3and 0.25 M Na2S mixed solution (pH = 12.5) under AM 1.5 G, 100 mW cm−2illumination. The V s -CIS-500 photoanode reveals the generation of photocurrent density higher than 5.0 mA cm −2 at 1.23 V vs. RHE without OER cocatalysts, which is superior to most of the other metal sulfide-based photoanodes (Supplementary Table 1 ) and also comparable to other up-to-date promising photoanodes, such as α-Fe 2 O 3 , BiVO 4 , and Ta 3 N 5 (Supplementary Table 2 ). The onset potential ( V on ) is determined by the intersection point of the J–V plot subtracting the contribution of the dark current curve (Supplementary Fig. 7 ). Noteworthily, the onset potential of the V s -CIS-500 photoanode (−148 mV) reveals a cathodic shift of 74 mV relative to that of CdIn 2 S 4 (−74 mV). The onset potential of the photoanode under illumination is generally influenced by two factors, i.e., the open-circuit photovoltage ( V ph ) and the kinetic overpotential ( η k ) as expressed by the following equation: E redox – V onset = V ph – η k , where E redox represents the electrochemical potential of the electrolyte solution that is irrelevant to the surface nature of the electrode [28] . Given that either an increase of V ph or a decrease of η k can give rise to the cathodic shift of E onset , confirming the crucial factor is of great importance to understand the effect of surface sulfur vacancies. The difference between the quasi-equilibrium under illumination and the equilibrium for CdIn 2 S 4 and V s -CIS-500 photoanodes is reported on the photovoltage (Fig. 2b , Supplementary Fig. 8 ). The difference of 78 mV between CdIn 2 S 4 and V s -CIS-500 photoanodes accounts for the above cathodic shift of 74 mV, illustrating that the increase of V ph rather than the decrease of η k is mainly responsible for the observed cathodic shift. Meanwhile, the equilibrium open-circuit potentials of both CdIn 2 S 4 (0.485 ± 0.003 V) and V s -CIS-500 (0.458 ± 0.004 V) photoanodes in the dark deviate from the ideal value (1.23 V), indicative of the significant potential drop within their Helmholtz layers [29] , which is detrimental to the photovoltage generation capabilities of CdIn 2 S 4 and V s -CIS-500 photoanodes. In principle, this adverse potential drop can be restrained by modification of co-catalysts [30] , [31] , which, however, is beyond the scope of this manuscript and will be discussed in our future work. The ABPE values derived from the J–V plots are also calculated (Eq. ( 2 )), and the V s -CIS-500 photoanode reveals a record-high value for single sulfide photon absorber to date (Fig. 2c ), achieving the maximum ABPE value of 2.49% at 0.477 V vs. RHE (Supplementary Table 1 ). Fig. 2: Photoelectrochemical performance. a Current–voltage ( J–V ) plots measured in 0.35 M Na 2 SO 3 and 0.25 M Na 2 S mixed solution (pH = 12.5) under dark and AM 1.5 G, 100 mW cm −2 illumination with a scan rate of 10 mV s −1 . b Open-circuit voltages of CdIn 2 S 4 and V s -CIS-500 photoanodes were recorded in 0.5 M Na 2 SO 4 solution (pH = 7) in the dark and under illumination. c ABPE measured with a two-electrode cell for water splitting in 0.35 M Na 2 SO 3 and 0.25 M Na 2 S mixed solution (pH = 12.5) under dark and AM 1.5 G, 100 mW cm −2 illumination. d IPCE measured at 0.6 V vs. RHE under monochromatic light irradiation. e SPV spectra of CdIn 2 S 4 and V s -CIS-500 nanoparticles. f Long-term stability test, as well as experimental and theoretical H 2 evolution, were measured in 0.35 M Na 2 SO 3 and 0.25 M Na 2 S mixed solution (pH = 12.5) under AM 1.5 G, 100 mW cm −2 illumination. Full size image Meanwhile, the incident photon-to-current conversion efficiencies (IPCE) under monochromatic light irradiation are also employed to illustrate the photoresponse of CdIn 2 S 4 and V s -CIS-500 photoanodes (Fig. 2d , Eq. ( 3 )), which reveals that the IPCE value is significantly improved in the light range of 350–500 nm, and the light to generate measurable photovoltage is truncated between 525 and 550 nm for the CdIn 2 S 4 photoanode while it extends up to ~650 nm for the V s -CIS-500 photoanode. To further verify whether the photocurrent enhancement is solely due to the improved photon absorption, we further calculate the absorbed photon-to-current efficiency (APCE, Supplementary Fig. 9 ), which manifests a significant enhancement in APCE for the V s -CIS-500 photoanode, particularly from 350 to 500 nm, indicating the improved efficiency in electron–hole separation. To further unravel the effect of surface sulfur vacancies on the electron–hole separation efficiency in the V s -CIS-500 photoanode, the surface photovoltage (SPV) spectroscopy was conducted (Fig. 2e ). The positive SPV spectra confirm the type of SS, that is, excitation of electrons from the SS to the conduction band [32] . Of note, except for the significantly increased photovoltage for the V s -CIS-500 photoanode which demonstrates its enhanced electron–hole separation, a broad peak is detected, and distinct sub-bandgap knees emerge, which is caused by both the Franz–Keldysh effect and photo-assisted charge transfer originated from shallow trap states [33] , also illustrative of the existence of trap states generated by sulfur vacancies. The PEC stability is examined by long-term photocurrent to time ( J – t ) measurement and the hydrogen evolution test at 0 V vs. Ag/AgCl reference electrode (Fig. 2f ). The J – t plot of V s -CIS-500 photoanode reveals no significant decay in the 15 h continued operation in 0.35 M Na 2 SO 3 and 0.25 M Na 2 S-mixed solution, illustrative of the stable characteristic of surface sulfur vacancies under illumination and applied bias. The XRD pattern, SEM image, and ESR signal of the V s -CIS-500 photoanode post-PEC test are further measured (Supplementary Fig. 10 ). No phase structural, morphological, and electronic structural changes are observed, indicative of its robust PEC stability. Besides, the XPS spectra of the V s -CIS-500 photoanode post-PEC test are also measured (Supplementary Fig. 11 ). The peak positions for Cd and In atoms are nearly unchanged, whereas the S 2 p orbital slightly shifts to higher binding energy and peaks that assigned to elemental sulfur appear, illustrative of oxidation reaction competing with the consumption rates of photoinduced carriers for water oxidation on the surface of V s -CIS-500 photoanode [34] , which suggests that the surface of V s -CIS-500 requires oxygen evolution catalysts (OECs) to form a stable V s -CIS-500/OEC interface to achieve long-term stability for photo-oxidation of water. Besides, the practical gas evolution in the Pt counter electrode is measured by gas chromatography (GC, Fig. 2f ). The hydrogen evolution rate of the V s -CIS-500 photoanode achieves a release rate of 89.2 μmol h −1 , which is ~5 times that of the pristine CdIn 2 S 4 photoanode and approaches its theoretical value (the dashed line). The Faradaic efficiency for hydrogen production measured at 0 V vs. Ag/AgCl reference electrode approaches 100% (Supplementary Fig. 12 ), also indicative of its high conversion efficiency. Furthermore, the PEC performance of the V s -CIS-500 photoanode without sacrificial agents are also investigated, revealing a current density of 4.76 mA cm −2 at 1.23 V vs. RHE and an ABPE value of 1.35% at 0.733 V vs. RHE (Supplementary Fig. 13 ), which are greatly enhanced compared with those of the pristine CdIn 2 S 4 photoanode and also comparable to other up-to-date promising photoanodes (Supplementary Table 2 ). However, the current density obviously decreases in 1 h continuous measurement in the 0.5 M Na 2 SO 4 solution, which also illustrates that surface modification of the V s -CIS-500 photoanode is necessary to stabilize the V s -CIS-500/electrolyte interface to achieve long-term stability. Optical and PEC characterizations for mechanism The strategies to improve the photoelectric conversion efficiency of the CdIn 2 S 4 photoanode follow the basic principles as in photocatalyst, that is, to achieve high photoabsorption ability ( J abs ), charge separation efficiency ( η se ) and injection efficiency ( η in ) [35] (Eq. ( 4 )). Thus, the increase of any term of them can contribute to the final improved PEC performance. To illustrate the effect of sulfur vacancies in the V s -CIS-500 photoanode and subsequently confirm the crucial factors for the improved PEC activity, we further measure the optical properties. The absorbance edge of V s -CIS-500 relative to that of CdIn 2 S 4 slightly extends from ~554 to ~579 nm, indicative of the small change in the bandgap. Meanwhile, the Urbach tail appears due to the shallow trap states generated by sulfur vacancies [36] (Fig. 3a ). The exact energy band structures of V s -CIS-500 are further determined by ultraviolet photoelectron spectroscopy (UPS) spectra and valence-band XPS spectra (Supplementary Fig. 14 ), which reveals few changes in the positions of valence band maximum (VBM), the conduction band minimum (CBM), and Fermi level ( E f ). Thus, we conclude that the shallow trap states generated by sulfur vacancies rather than the changes of the intrinsic band positions are the critical factors to improve PEC activity. To further elucidate the effect of surface sulfur vacancies, the photon absorption rates of CdIn 2 S 4 and V s -CIS-500 photoanodes are calculated (Supplementary Fig. 15 , Eq. ( 5 )), and the J abs value of V s -CIS-500 does not reveal much enhancement relative to that of CdIn 2 S 4 , which illustrates that introducing sulfur vacancies cannot improve light harvesting and J abs is not the crucial factor for the boosted photocurrent density. The η se is related to the photoinduced electron–hole separation, while the η in is related to the electron–hole recombination on their surfaces [37] . Both the values of η se and η in are significantly improved in the V s -CIS-500 photoanode relative to those in the CdIn 2 S 4 photoanode (Fig. 3b, c , Eqs. ( 6 ) and ( 7 )), illustrating that the more efficient photoinduced electron–hole separation and holes transferring to the surface after introducing of surface sulfur vacancies. Thus, the sulfur vacancies mainly account for the improved η se and η in , which are also crucial factors to the boosted photocurrent. Fig. 3: Optical and photoelectrochemical characterizations. a UV–vis diffuse reflectance spectra. b Charge separation efficiency and c charge injection efficiency vs. potential curves. d Steady-state PL spectra with excitation wavelength λ ex = 370 nm. e Time-resolved transient PL decay spectra with excitation wavelength λ ex = 370 nm. Inset is the fitted results according to a tri-exponential model, \(I\left( t \right) = \sum\nolimits_{i = 1}^{i = 3} {A_i{\mathrm{{e}}}^{ - t/\tau _i}}\) , where I ( t ), τ i, and A i were the intensity, the lifetime, and the amplitude of the i th component, respectively. f PALS of CdIn 2 S 4 and V s -CIS-500. Inset is the fitted results according to the following equation, \(N\left( t \right) = \mathop {\sum}\nolimits_{{\mathop{i}\nolimits} = 1}^{{\mathop{k}\nolimits} + 1} {\frac{{I_{\mathrm{i}}}}{{\tau _i}}\exp \left( { - \frac{t}{{\tau _i}}} \right)}\) , where τ 1 , τ 2 , τ 3 were three positron lifetime components, and I 1 , I 2 I 3 were corresponding to the relative intensities. Full size image Moreover, the efficiency of charge separation is investigated by steady-state photoluminescence (PL) spectra (Fig. 3d ), and a broad emission peak derived from band-to-band transition is observed at ca. 549 nm. The lower PL peak intensity of V s -CIS-500 also illustrates its suppressed photoinduced charge recombination that is probably arising from the enhanced charge transport. More importantly, the reduced PL intensity of V s -CIS-500 demonstrates that the shallow trap states introduced by sulfur vacancies facilitate the photoinduced charge carrier separation rather than recombination. The charge carrier lifetimes of CdIn 2 S 4 and V s -CIS-500 are further evaluated by time-resolved photoluminescence (TRPL) spectra (Fig. 3e ). The PL decay can be well fitted to a tri-exponential model, and the V s -CIS-500 manifests a longer average lifetime (40.67 ns) than CdIn 2 S 4 (21.78 ns), indicating that more photoinduced electrons and holes can participate in the reaction for V s -CIS-500. Simultaneously, the lifetime of bulk and surface defects can be directly measured by positron annihilation lifetime spectra (PALS) (Fig. 3f ). The lifetime components τ 1 and τ 2 correspond to positrons captured by bulk defects and surface defects, respectively [38] . The values of τ 1 and τ 2 for V s -CIS-500 alter little compared with those of CdIn 2 S 4 , indicative of their similar characteristics for surface and bulk defects [39] . Moreover, The value of I 2 / I 1 that reflects the intensity ratio of surface to bulk defects is calculated to be 4.07 for V s -CIS-500, obviously higher than the 2.68 of pristine CdIn 2 S 4 , which directly demonstrates that the enhanced surface-deficient density is ascribed to the introduction of sulfur surface vacancies. Charge transfer and recombination kinetics To more clearly illustrate charge recombination and transfer kinetics, we further investigate the interfacial kinetics of CdIn 2 S 4 and V s -CIS-500 photoanodes. There are two different mechanisms for possible hole transfer routes, that is, direct hole transfer from valence band or indirect hole transfer by trapping holes at SS (Supplementary Fig. 16 ), and the route transferred through SS are recognized as the predominant route, whose density of states (DOS) is proportional to the photocurrent density [40] . Therefore, we employ the electrochemical impedance spectroscopy (EIS) to incisively illustrate changes of the resistances and capacitances that are associated with the charge trapping ( R trapping , C bulk ) and transfer ( R ct, trap , C trap ) at/from SS. The values for the charge trapping and transfer parameters are extracted from the fitted EIS plots according to the corresponding equivalent circuit [41] (see details in Supplementary Fig. 17 ). The significant enhanced C bulk value for V s -CIS-500 indicates the increased carrier density after introducing sulfur vacancies in the depletion layer (Fig. 4a ), which is consistent with the DOS calculation (Fig. 1g ), and the decreased R trapping value for V s -CIS-500 illustrates the recombination of photoinduced electrons and holes are much restrained. Meanwhile, the correlation between the increase of C trap and the decrease of R ct, trap for the V s -CIS-500 photoanode confirms that the photo-oxidation indeed occurs from the SS as reported in other works [42] , [43] . Moreover, compared with the CdIn 2 S 4 photoanode, the V s -CIS-500 photoanode reveals more drastic changes in C trap rather than in C bulk , illustrative of the role of the sulfur vacancies mainly embodied in improving the DOS of SS and reducing the transfer resistance of holes to the water, instead of enhancing the charge recombination. The DOS of SS is further derived from the C trap on the basis of the following relationship: N ss ( E ) = C trap ( E )/ q , where N ss ( E ) is the DOS of SS as a function of potential, and q is the elementary charge [44] . The SS energy distribution follows a Gaussian curve located below the photocurrent onset with its Fermi level pinned at SS (Fig. 4b ). The restrained SS distribution and the positive shift of the DOS center of the V s -CIS-500 photoanode are the thermodynamically fundamental reasons for the larger V ph and also account for its high photocurrent density. Besides, the charge carrier density in the space charge region for V s -CIS-500 (9.94 × 10 20 cm −3 ) is significantly increased compared to that of CdIn 2 S 4 (1.02 × 10 19 cm −3 ), as derived from the Mott–Schottky plots (Fig. 4c , Eq. ( 9 )), which evidences the boosted charge transfer, also in accordance with earlier the DOS calculation for V s -CIS-500 with S 3 p shallow trap states to accumulate more charge carriers (Fig. 1g ). Notably, a negative shift of the flat band potential for the V s -CIS-500 photoanode is observed, which illustrates the sharper band bending between V s -CIS-500 photoanode and electrolyte. Here, the sulfur vacancy with a 2+ charge state has the lowest formation energy according to the DFT calculation. Therefore, the surface sulfur vacancy becomes positively charged \({\mathop{\rm{S}}\nolimits} _{\mathrm{{{vac}}}}^{2 + }\) and donates free carriers to the conduction band of CdIn 2 S 4 as in other refs. [45] , [46] , resulting in the significant increase of the charge carrier density at the surface region. Recent research illustrates that increasing the carrier density provides an effective method to shorten the depletion width ( W d ) and enhance the band bending for hole collection [23] . The W d of CdIn 2 S 4 photoanode dramatically decreases from 8.5 to 0.9 nm after introducing surface sulfur vacancies at 1.23 V vs. RHE (Eq. ( 10 )), which indicates a sharper band bending at the V s -CIS-500/electrolyte interface, resulting in the acceleration of hole drift from depletion region to surface and the suppression of the charge recombination. Therefore, the shortening of the depletion width and enhanced charge separation in V s -CIS-500 photoanode after introducing surface sulfur vacancies is responsible for the improved photocurrent. Fig. 4: Charge transfer and recombination kinetics. a Capacitances and resistances parameters associated with the charge trapping ( R trapping , C bulk ) and transfer ( R ct, trap , C trap ) at/from surface states with different applied potentials that are determined from the EIS spectra. Among others, the R s is defined as the series resistance in the PEC cell, C bulk represents the capacitance of charge accumulation in the space charge layer, R trapping represents the resistance of holes trapping at the surface states, R ct, bulk represents the resistance of holes directly transferred from valence band to conduction band, R ct, trap represents the resistance of charge transfer from the surface states to the solution, and C trap represents the capacitance associated with charge accumulation on the surface states. b DOS of surface states (SS) as a function of applied potential for CdIn 2 S 4 and V s -CIS-500 photoanode derived from the C trap . The lines are fitted by a Gaussian model. c Mott–Schottky plots. d IMPS spectra of the CdIn 2 S 4 and V s -CIS-500 photoanodes under the applied bias of 1.13 V. e The plot of the rate constant of charge transfer vs. potential. f The plot of the rate constant of charge recombination vs. potential. Full size image To directly grasp the behavior of photoinduced charge carriers across the Helmholtz layer, we employ intensity-modulated photocurrent spectroscopy (IMPS) to evaluate the pseudo-first-order rate constants of hole transfer ( k tran ) and surface recombination ( k rec ) [47] . As depicted in Fig. 4d , both the recombination (upper quadrant semicircle) and RC attenuation (lower quadrant semicircle) are quite different between CdIn 2 S 4 and V s -CIS-500 photoanodes. The average photoinduced electron transfer time ( τ d ) estimated from the frequency at the minimum imaginary part (Eq. ( 11 )) reveals that the τ d for the V s -CIS-500 photoanode is much shorter compared to that of CdIn 2 S 4 (Supplementary Fig. 18 ), suggesting its superior charge transfer rate. Moreover, the IMPS spectra at different applied bias are further measured to deduce the values of k tran and k rec (Supplementary Fig. 19 ), and the V s -CIS-500 photoanode manifests an increase in k tran and a decrease in k rec (Eqs. ( 12 )–( 13 )) compared to the CdIn 2 S 4 photoanode (Fig. 4e, f ), which are the quantitative evidence for the enhanced hole transfer rate and suppressed surface recombination rate across the Helmholtz layer, and consequently accounts for improved photocurrent density in kinetics. DFT calculations The effect of surface sulfur vacancies on the interfacial OER process was investigated using DFT calculations to elucidate the potential-determining step. Considering that the hole scavengers, that is, H 2 O molecules in the neutral electrolyte must initially absorb on the active site of CdIn 2 S 4 and V s -CdIn 2 S 4 photoanodes to accomplish the following OER steps, the adsorption energy of H 2 O molecules is calculated in consequence. The adsorption energies are determined to be −1.251, and −0.425 eV for CdIn 2 S 4 and V s -CdIn 2 S 4 (Supplementary Note 3 ), respectively, which indicates decomposition of H 2 O molecules to generate OER intermediates on V s -CdIn 2 S 4 is more favorable according to the Sabatier principle [48] . Furthermore, the evolution of three intermediates, OH*, O*, and OOH* involved in the OER processes is further calculated in terms of Gibbs free energy. Interestingly, the stable absorbing geometries of intermediates for V s -CdIn 2 S 4 reveal that all the terminal O atoms coordinate with adjacent three In atoms, which is just the location of sulfur vacancy (Supplementary Fig. 26 ). It confirms the earlier difference charge density calculation result, which manifests the charge accumulation on the adjacent Cd and In atoms (Fig. 1h ) after introducing surface sulfur vacancies, beneficial to chemisorption of the OER intermediates. Moreover, the largest Gibbs free energy difference (Fig. 5a , Δ G 3 = 2.418 V, corresponding to η OER = 1.123 V) for pristine CdIn 2 S 4 occurs in the process of formation of OOH* from O*, which illustrates that the strong adsorption of OOH* on CdIn 2 S 4 is the potential-determining step in the OER process. Besides, despite the unchanged potential-determining step in V s -CdIn 2 S 4 (Fig. 5b ), the Gibbs free energy is decreased to 2.064 V, resulting in η OER remarkably reducing to 0.834 V. The change for the theoretical η OER agrees with the experimental overpotentials determined by J – V curves without illumination (Supplementary Fig. 20 ), which illustrates that the surface sulfur vacancies reduce the OER overpotential by lowing the formation of OOH*. Notably, the negative Gibbs free energy for the formation of OH* in V s -CdIn 2 S 4 without applied bias illustrates that the formation of OH* is a thermodynamically favorable process, indicative of the location of surface sulfur vacancies easily occupied by OH*, which prevents the possible self-oxidation due to the high oxidation potential of photoinduced holes and ensures the stability of this sulfide photoanode. Fig. 5: OER mechanism for the CdIn 2 S 4 photoanode. a Free energies of OER steps for CdIn 2 S 4 ( \(0\overline 1 1\) ). b Free energies of OER steps for V s -CdIn 2 S 4 ( \(0\overline 1 1\) ). c Comparison of density of states for V s -CdIn 2 S 4 ( \(0\overline 1 1\) ) without applied bias and with an applied bias of 1.23 V. d Photoexcited charge-transition route change for V s -CdIn 2 S 4 ( \(0\overline 1 1\) ) from HOMO states (in the range of 0–0.5 eV below the Fermi level) to LUMO states (in the range of 0–1 eV above the Fermi level) with an applied bias of 1.23 V (isosurface set at 0.004e Bohr −3 ). The charge difference density is calculated by Δ ρ = ρ 1.23V − ρ 0V , and the yellow region represents electron accumulation. Full size image Given the implementation of applied bias in practical PEC tests, the band structure of V s -CdIn 2 S 4 may be changed under applied bias, reflected in the shifts of Fermi level and band offsets in the interfacial region [49] , [50] . Therefore, the effect of applied bias on the band structure of V s -CdIn 2 S 4 is also taken into account. As depicted in Fig. 5c , the Fermi level, and bandgap for V s -CdIn 2 S 4 reveal little changes after imposing a bias of 1.23 V, which demonstrates little influence of applied bias on the intrinsic band structure of V s -CdIn 2 S 4 , further illustrative of the main reason for the improved photocurrent due to the trap states generated by sulfur vacancies. To further unravel the effect of trap states on the charge-transfer routes under the applied bias, photoexcited charge density transition from the sulfur vacancy-induced hybrid highest occupied molecular orbital (HOMO) states to the lowest unoccupied molecular orbital (LUMO) are investigated. As revealed in Fig. 5d , the charge densities of the hybrid HOMO states are nearly unchanged while the charge densities of the hybrid LUMO states are obviously increased in the adjacent In and Cd atoms of sulfur vacancies as indicated by the arrow, illustrative of more charge density generated in the energy range of Fermi level to the LUMO states to facilitate the charge separation and transfer, which is considered to be the reason for the enhanced photocurrent density with the increase of applied bias for the V s -CIS-500 photoanode. In summary, we have developed a highly active, deficient ternary sulfide (CdIn 2 S 4 ) photoanode for PEC water splitting. The surface sulfur vacancies in CdIn 2 S 4 are mainly responsible for the improved photocurrent. The effects of surface sulfur vacancies are thoroughly investigated by theoretical calculations and experimental characterizations. The theoretical calculations suggest that introduced surface sulfur vacancies bring about charge accumulation on the adjacent In and Cd atoms, which become the active sites for OER intermediates, resulting in the decreased potential in the rate-determining step. The optical characterizations demonstrate the dominant effects of the surface sulfur vacancies on charge separation and injection efficiencies, indicative of the shallow trap states introduced by sulfur vacancies facilitating the charge separation and transfer. The characterizations of kinetics about charge transfer and recombination further confirmed the improved hole transfer rate and suppressed surface charge recombination in the SS, which are the fundamental reasons for the enhanced photocurrent. Benefiting from the surface sulfur vacancies, the CdIn 2 S 4 photoanode reveals a photocurrent density of 5.73 mA cm −2 at 1.23 V vs. RHE and an ABPE value of 2.49% at 0.477 V vs. RHE, which make it a promising candidate for PEC water splitting. Synthesis of the CdIn 2 S 4 photoanode The fluorine-doped tin oxide conductive glasses (FTO, 10 Ω sq −1 ) were pretreated by successive sonication in acetone, ethanol, and distilled water. In a typical procedure, stoichiometric amounts of Cd(NO 3 ) 2 ·4H 2 O (0.6 mmol), In(NO 3 ) 3 ·5H 2 O (1.2 mmol), and excessive amounts of thioacetamide (CH 3 CSNH 2 ) (9.6 mmol) were dissolved in 35 mL of distilled water (Milli-Q) and then transferred into a 50 mL Teflon-lined stainless autoclave. Subsequently, the pretreated FTO was placed at an angle against the wall of the Teflon-liner with the conductive side facing down. The autoclave was sealed and maintained at 160 °C for 10 h, followed by cooling naturally to room temperature. Finally, the FTO substrate deposited with CdIn 2 S 4 film was rinsed with distilled water and dried in air at room temperature. Synthesis of the V s -CIS photoanode In a typical procedure, the as-synthesized CdIn 2 S 4 photoanode was annealed for 2 h under H 2 /Ar-mixed gas flux (1:10 vol/vol, 100 mL min −1 ) atmosphere at a temperature of 350–550 °C with a heating rate of 5 °C min −1 . After cooling naturally to room temperature, the V s -CIS photoanode was obtained and denoted as V s -CIS- T ( T refers to the annealing temperature). Characterizations PXRD patterns were collected on a Bruker AXS D8 diffractometer in the Bragg–Brentano mode, using Cu Kα radiation (1.5418 Å). The morphology and microstructure of the samples were investigated by transmission electron microscopy (TEM, JEOL JEM-1011) and field-emission scanning electron microscopy (FE-SEM, SU8010). The lattice structures were observed by high-resolution transmission electron microscopy (HRTEM, JEOL JEM-2100) and spherical aberration-corrected TEM (Titan Cubed Themis G2 300). The XPS and valence-band XPS (VB-XPS) were recorded on a Thermo scientific ESCALAB 250Xi with 30.0 eV pass energy and an Al Kα line excitation source, using C 1 s (binding energy of 284.8 eV) as a reference. The UPS was conducted with a monochromatic He light source (21.22 eV), and a bias of 8 eV was applied to observe the secondary electron cutoff edge. The optical properties of samples were investigated by an ultraviolet–visible spectrophotometer (Cary 100, Agilent Technologies). The PL spectra (excited by 370 nm light illumination) were measured using a fluorescence spectrophotometer (G9800A, Agilent Technologies). The TRPL spectroscopy under the excitation of 377.8 nm laser was performed on a fluorescence lifetime spectrophotometer (FLS920, Edinburgh). The ESR spectra were recorded on a spectrometer (JES-X320, JEOL) at 300 K and 9165.365 MHz. SPV spectroscopy was carried out on the basis of a lock-in amplifier to study the separation characteristics of the photogenerated charges by the spectrometer (CEL-SPS1000, Ceaulight Technology Co. Ltd., China). PEC property measurements PEC measurements were carried out on an electrochemical workstation (CHI 760e, CH Instruments Inc., China) at room temperature with a conventional three-electrode cell. The prepared photoanode with an exposed area of 1 × 1 cm 2 was employed as the working electrode, while the saturated Ag/AgCl electrode and Pt foil were used as the reference electrode and counter electrode, respectively. A 300 W xenon arc lamp (CEL-PE300L-3A) with a filter (AM 1.5 G, Ceaulight Technology Co. Ltd., China) was employed to simulate solar illumination with about 1 Sun power. The back-side illumination through the FTO side was adopted for all the PEC tests. The photo-oxidation of sulfite performance was measured in a 0.35 M Na 2 SO 3 and 0.25 M Na 2 S-mixed solution (pH = 12.5), while the photo-oxidation of water performance was measured in a 0.5 M Na 2 SO 4 solution (pH = 7). To study the kinetics of charge transfer and recombination, 0.5 M Na 2 SO 4 solution (pH = 7) was used as the electrolyte. The amounts of evolved H 2 and O 2 were determined at regular time intervals using GC (3420A, Beifen-Ruili Co. Ltd., China) with a thermal conductivity detector and a 5 Å molecular sieve column. During the evaluation of the PEC performance of CdIn 2 S 4 and V s -CIS photoanodes, all measured potentials were converted to reversible hydrogen electrode (RHE) using the Nernst equation below. E_RHE = E_Ag/AgCl + E_Ag/AgCl( reference) + 0.0591  1ptV×pH
 (1) ( E Ag/AgCl (reference) = 0.1976 V vs. NHE at 25 °C) The ABPE was calculated from the J–V curve using the equation [51] : 
    ABPE = [ j_ph( mA 1pt cm^ - 2) ×( 1.23 - V_bias)( V)/P_total( mW  1ptcm^ - 2)]_AM1.5G
 (2) where j ph is the photocurrent density obtained under an applied bias ( V bias ), and P total is the incident illumination power density. The IPCE at different wavelengths was measured at 0.6 V vs. RHE using monochromatic light illumination from a 300 W Xe arc lamp equipped with a monochromator (CEL-QPCE3000, Ceaulight Technology Co. Ltd., China). The IPCE values were determined using the equation [51] : 
    IPCE( λ) = j_ph( mA  1ptcm^ - 2) × 1239.8( V×nm)/P_mono( mW  1ptcm^ - 2) ×λ( nm)
 (3) where 1239.8 V nm represents a multiplication of h (Planck’s constant) and c (the speed of light), λ is the incident light wavelength (nm), and P mono is the monochromated illumination power intensity. Supplemented equations for evaluating photocurrent density 
    J_ph = J_abs×η_seperation×η_injection
 (4) 
    J_abs = q/hc∫_λλϕ _λη_absdλ
 (5) 
    η_seperation = J_ph^Na_2SO_3/Na_2S/J_abs
 (6) 
    η_injection = J_ph^Na_2SO_4/J_ph^Na_2SO_3/Na_2S
 (7) 
    η_abs = ( 1 - 10^ - A) × 100%
 (8) The \({\it{J}}_{{\mathrm{ph}}}^{{{{\rm{Na}}_2{\rm{SO}}_3/{\rm{Na}}_2{\rm{S}}}}}\) is the photocurrent density measured in 0.35 M Na 2 SO 3 and 0.25 M Na 2 S mixed electrolyte, which serves as hole scavengers and ensures the hole injection rate approaching 100%, and \({\it{J}}_{{\mathrm{ph}}}^{{{{\rm{Na}}_2{\rm{SO}}_4}}}\) is the photocurrent densities measured in 0.5 M Na 2 SO 4 . The J abs is the photon adsorption rate expressed as the photocurrent density, and q is the charge of an electron, h is the Plank constant, c is the light speed, ϕ λ is the photon flux of the AM 1.5 G solar spectrum, and η abs is the light absorption efficiency [52] . Measurement of Mott–Schottky plots The charge carrier density in the space charge region was measured in a 0.5 M Na 2 SO 4 solution at a frequency of 1 kHz in the dark, and calculated according to the Mott–Schottky equation [53] 
    1/C^2 = 2/εε_0A^2qN_D×( V - V_fb - k_BT/q)
 (9) where C is the space-charge capacitance, V ( V vs. RHE) is the applied voltage, V fb ( V vs. RHE) is the flat-band potential, N D is the charge carrier density, ε is the dielectric constant of the semiconductor (taken as 6.6 for the CdIn 2 S 4 [54] ), ε 0 is the vacuum permittivity (8.854 × 10 −12 C V −1 m −1 ), k B is Boltzmann’s constant (1.381 × 10 −23 J K −1 ), q is the electronic charge (1.602 × 10 −19 C), and T is the absolute temperature. The thickness of the depletion width ( W d ) can be calculated as [55] 
    W_d = [ 2ε _oε( V - V_fb)/qN_D]^1/2
 (10) IMPS and PEIS measurements The IMPS and PEC impedance spectroscopy (PEIS) measurements were conducted on an electrochemical workstation (CIMPS-Pro, Zahner Co.) in 0.5 M Na 2 SO 4 solution with a three-electrode configuration at different bias potentials. For the IMPS measurement, modulated illumination was provided by a high-intensity light-emitting diode (LED: LSW-2) controlled by a LED driver (PP211) that allowed the superimposition of sinusoidal modulation (~10%) on a dc illumination level. The wavelength of light was 430–720 nm in the visible light region with an average intensity of 100 mW cm −2 . The modulation amplitude of the lamp voltage was 100 mV. The photocurrent as a function of frequency (from 0.1 to 10 kHz) after the light turned on was recorded. In the typical IMPS response, the average photogenerated electron transfer time ( τ d ) can be estimated from the frequency at the minimum imaginary part [56] 
    τ _d = 1/2π f_min
 (11) The frequency at the maximum imaginary part corresponds to the sum of the charge transfer ( k tran ) and recombination ( k rec ) rate constants as expressed [56] 
    k_tran + k_rec = 2π f_max
 (12) The hole transfer efficiency ( η tran ) at the semiconductor/electrolyte interface can be determined by the ratio of the steady-state photocurrent ( j ss ) to the instantaneous photocurrent ( j hole ). Assuming that both hole transfer and recombination are pseudo-first-order in the surface hole concentration, the hole transfer efficiency can also be expressed by the ratio of k rec and k tran [57] 
    η _tran = j_ss/j_hole = k_tran/k_tran + k_rec
 (13) The PEIS measurements were carried out in a frequency range of 0.1 Hz to 100 kHz with an amplitude of 5 mV under constant light (430–720 nm, 100 mW cm −2 ) illumination. The Randles equivalent circuit was used to analyze the impedance data using Zview software (Scribner Associates). PALS measurement PALS measurements were carried out with a fast–fast coincidence system with a time resolution of 190 ps full width at half-maximum (FWHM) for the γ -rays from a 60 Co source selected under the experimental conditions. The sample powder was pressed into a disk (diameter: 10.0 mm, thickness: 1.0 mm). A 4 × 10 5 Bq source of 22 Na was sandwiched between two identical sample disks. The positron lifetime spectrum containing 2 × 10 6 counts were analyzed by the computer program Limetime9.0 to decompose several lifetime components. DFT calculations for surface energy The first-principle calculations corrected by on-site Coulomb interaction were carried out with the Vienna ab initio simulation package (VASP) [58] , [59] . The interaction between ions and valence electrons was described using the projector-augmented wave (PAW) potentials, and the exchange-correction function was treated using the generalized gradient approximation (GGA) in the Perdew–Burke–Ernzerhof for solid (PBEsol) form [60] . Interactions between the valence electrons and the ion core are represented in 4 d 10 5 s 2 , 4 d 10 5 s 2 5 p 1 , and 3 s 2 3 p 4 orbitals for Cd, In and S, respectively. The wave functions were expanded in a plane wave basis with an energy cutoff of 500 eV, which was high enough to ensure that no Pulay stresses occur within the cell during geometry relaxation. The effective U–J values of 2.1 and 1.9 were employed to account for the strong on-site Coulomb interaction of Cd and In atoms [61] , respectively. The Brillouin zone was sampled by a Γ-centered method, and a K-points resolved value of 0.02 was employed for all the geometries optimization, which was set to 0.01 for the density of states calculations. The Fermi level was slightly broadened using Fermi–Dirac smearing of 50 meV. For all the calculations, the convergence criteria for the electronic and ionic relaxation are 10 −5 eV and 0.02 eV/Å, respectively. Based on the BFDH theory and the experimental morphology of CdIn 2 S 4 (Fig. 1e ), we constructed the geometry of CdIn 2 S 4 , which was consisted of {100}, {110}, and { \(0\overline 1 1\) } family of crystal planes. Given the effect of truncated atoms on the surface energy, (100), (110), and ( \(0\overline 1 1\) ) crystal planes with variable truncated atoms were taken into account. The symmetrical slab models with a vacuum thickness of 30 Å were adopted to simulate the geometries of possible exposed planes (Supplementary Fig. 21 ), and the surface energies in their possible chemical potentials were calculated according to the following equation: 
    γ = 1/2A( E_s^relax - n_Cdμ _Cd - n_Inμ _In - n_Sμ _S)
 (14) where A is the surface area, \(E_{\mathrm{{s}}}^{{\mathrm{{relax}}}}\) is the total energy of the relaxed slab, and n Cd , n In , and n S are the numbers of Cd, In, and S involved in the slab model, μ Cd , μ In , and μ S are the atomic chemical potential of Cd, In, and S atoms, respectively. The factor of 1/2 corresponded to two equivalent surfaces in the slab models (see details in Supplementary Fig. 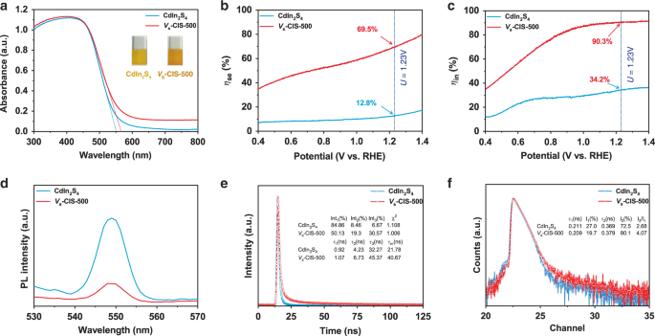Fig. 3: Optical and photoelectrochemical characterizations. aUV–vis diffuse reflectance spectra.bCharge separation efficiency andccharge injection efficiency vs. potential curves.dSteady-state PL spectra with excitation wavelengthλex= 370 nm.eTime-resolved transient PL decay spectra with excitation wavelengthλex= 370 nm. Inset is the fitted results according to a tri-exponential model,\(I\left( t \right) = \sum\nolimits_{i = 1}^{i = 3} {A_i{\mathrm{{e}}}^{ - t/\tau _i}}\), whereI(t),τi,andAiwere the intensity, the lifetime, and the amplitude of theithcomponent, respectively.fPALS of CdIn2S4andVs-CIS-500. Inset is the fitted results according to the following equation,\(N\left( t \right) = \mathop {\sum}\nolimits_{{\mathop{i}\nolimits} = 1}^{{\mathop{k}\nolimits} + 1} {\frac{{I_{\mathrm{i}}}}{{\tau _i}}\exp \left( { - \frac{t}{{\tau _i}}} \right)}\), whereτ1, τ2, τ3were three positron lifetime components, andI1,I2I3were corresponding to the relative intensities. S22 and Supplementary Table 3 ). DFT calculations for the sulfur vacancy To illustrate the most feasible plane for the formation of surface sulfur vacancy, slabs models with vacuum thickness of 15 Å were constructed, as shown in Supplementary Fig. 23 . To minimize the effect of spurious electrostatic interactions in charged defect calculations due to the periodic cell approximation, a 2 × 2 periodic surfaces were employed to ensure the distance of the sulfur vacancies in adjacent cells over 10 Å. The bottom atoms were saturated with H and pseudo-potential 0.5H to remove the dangling bonds. The possibility of production of the surface sulfur vacancy in (100), (110), and ( \(0\overline 1 1\) ) crystal planes was evaluated by the formation energy which is estimated as [62] , 
    Δ H_f( X^q) = E_tot( X ^q) - E_tot( bulk) - ∑_in_iμ _i + q( E_v + E_F)
 (15) where E tot ( X q ) and E tot (bulk) are the total energies of the defect X with charge q and bulk, respectively. The n i is the number of atoms being added to ( n i > 0) and/or removed from ( n i < 0) in the perfect-crystal supercell, and μ i is the atomic chemical potential. E VBM is the energy of the valence-band maximum (VBM), and E F is the Fermi level measured from the VBM, varying in the range of the bandgap E g (see details in Supplementary Fig. 24 and Supplementary Fig. 25 ). 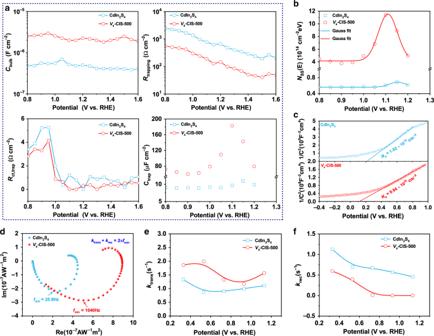Fig. 4: Charge transfer and recombination kinetics. aCapacitances and resistances parameters associated with the charge trapping (Rtrapping,Cbulk) and transfer (Rct, trap,Ctrap) at/from surface states with different applied potentials that are determined from the EIS spectra. Among others, theRsis defined as the series resistance in the PEC cell,Cbulkrepresents the capacitance of charge accumulation in the space charge layer,Rtrappingrepresents the resistance of holes trapping at the surface states,Rct, bulkrepresents the resistance of holes directly transferred from valence band to conduction band,Rct, traprepresents the resistance of charge transfer from the surface states to the solution, andCtraprepresents the capacitance associated with charge accumulation on the surface states.bDOS of surface states (SS) as a function of applied potential for CdIn2S4andVs-CIS-500 photoanode derived from theCtrap. The lines are fitted by a Gaussian model.cMott–Schottky plots.dIMPS spectra of the CdIn2S4andVs-CIS-500 photoanodes under the applied bias of 1.13 V.eThe plot of the rate constant of charge transfer vs. potential.fThe plot of the rate constant of charge recombination vs. potential. 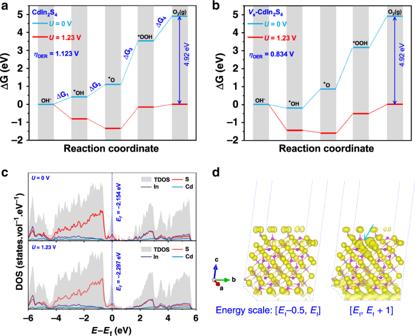Fig. 5: OER mechanism for the CdIn2S4photoanode. aFree energies of OER steps for CdIn2S4(\(0\overline 1 1\)).bFree energies of OER steps forVs-CdIn2S4(\(0\overline 1 1\)).cComparison of density of states forVs-CdIn2S4(\(0\overline 1 1\)) without applied bias and with an applied bias of 1.23 V.dPhotoexcited charge-transition route change forVs-CdIn2S4(\(0\overline 1 1\)) from HOMO states (in the range of 0–0.5 eV below the Fermi level) to LUMO states (in the range of 0–1 eV above the Fermi level) with an applied bias of 1.23 V (isosurface set at 0.004e Bohr−3). The charge difference density is calculated by Δρ=ρ1.23V−ρ0V, and the yellow region represents electron accumulation. DFT calculations for surface OER mechanism The slab models of ( \(0\overline 1 1\) ) planes with In and S as truncated atoms were constructed to elucidate the potential-determining step in surface OER process by calculating the evolution of OH*, O*, and OOH* intermediates on CdIn 2 S 4 and deficient CdIn 2 S 4 . As shown in Supplementary Fig. 26 , the slab model consisted of eight atomic layers and a vacuum thickness of 15 Å. Similarly, the bottom atoms were saturated with H and pseudo-potential 0.5H to remove the dangling bonds (see details in Supplementary Note 3 ).